Suppression of spin-bath dynamics for improved coherence of multi-spin-qubit systems Multi-qubit systems are crucial for the advancement and application of quantum science. Such systems require maintaining long coherence times while increasing the number of qubits available for coherent manipulation. For solid-state spin systems, qubit coherence is closely related to fundamental questions of many-body spin dynamics. Here we apply a coherent spectroscopic technique to characterize the dynamics of the composite solid-state spin environment of nitrogen-vacancy colour centres in room temperature diamond. We identify a possible new mechanism in diamond for suppression of electronic spin-bath dynamics in the presence of a nuclear spin bath of sufficient concentration. This suppression enhances the efficacy of dynamical decoupling techniques, resulting in increased coherence times for multi-spin-qubit systems, thus paving the way for applications in quantum information, sensing and metrology. Understanding and controlling the coherence of multi-spin-qubit solid-state systems is crucial for quantum information science [1] , [2] , [3] , basic research on quantum many-body dynamics [4] and quantum sensing and metrology [5] , [6] , [7] , [8] , [9] . Examples of such systems include nitrogen-vacancy (NV) colour centres in diamond [10] , phosphorous donors in silicon [11] and quantum dots [12] . In characterizing the potential usefulness of multi-qubit systems for quantum applications, the product of the qubit density ( n qb ) and the qubit coherence lifetime ( T 2 ) serves as a basic figure-of-merit (FOM), FOM= n qb T 2 . For example, in quantum measurements the phase-shift sensitivity δφ scales as [5] , [13] , [14] , [15] . Increasing this multi-qubit FOM requires an understanding of the sources of decoherence in the system and their interplay with qubit density. In particular, for solid-state spin qubits T 2 is typically limited by interaction with an environment (that is, bath) of paramagnetic spin impurities, whereas n qb is limited by fabrication issues, the associated creation of additional spin impurities in the environment, and the ability to polarize (state prepare) the quantum spins. The paradigm of a central spin coupled to a spin environment has been studied intensively for many years (see for example refs 16 and 17 ), and quantum control methods have been developed to extend the spin coherence lifetime by reducing the effective interaction with the environment. In particular, dynamical decoupling techniques pioneered in nuclear magnetic resonance have recently been applied successfully to extend the effective T 2 of single NV-diamond electronic spins by more than an order of magnitude [18] , [19] , [20] . Here we study experimentally the spin environment of NV colour centres in room temperature diamond and their multi-spin-qubit FOM. We apply a spectral decomposition technique [21] , [22] , [23] to characterize the dynamics of the composite solid-state spin bath, consisting of both electronic spin (N) and nuclear spin ( 13 C) impurities. We study three different diamond samples with a wide range of NV densities and impurity spin concentrations (measuring both NV ensembles and single NV centres), and find unexpectedly long correlation times for the electronic spin baths in two diamond samples with natural abundance (1.1%) of 13 C nuclear spin impurities. We identify a possible new mechanism in diamond involving an interplay between the electronic and nuclear spin baths that can explain the observed suppression of electronic spin-bath dynamics. We show that this spin-bath suppression enhances the efficacy of dynamical decoupling techniques, enabling large values for the multi-qubit FOM ~2×10 14 (ms cm −3 ; compare, for example, to ref. 24 , and to the similar FOM obtained with a much higher NV density sample [9] ). Spectral decomposition technique Owing to coupling of the NV spins to their magnetic environment ( Fig. 1a,b ), coherence is lost over time with the general form C ( t )= e − χ ( t ) , where the functional χ ( t ) describes the time dependence of the decoherence process ( Supplementary Methods ). In the presence of a modulation acting on the NV spins (for example, a resonant MW (microwave) pulse sequence), described by a filter function in the frequency domain F t ( ω ) (see below), the decoherence functional is given by [25] , [26] . 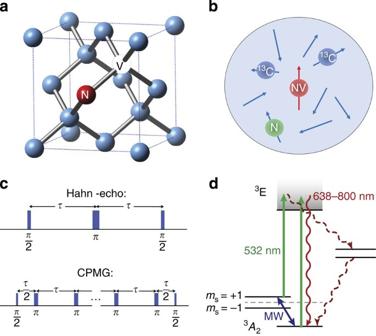Figure 1: NV centre in diamond and applied spin-control pulse sequences. (a) Lattice structure of diamond with an NV colour centre. The NV electronic spin axis is defined by nitrogen and vacancy sites, in one of four crystallographic directions in the diamond lattice. NV orientation subsets can be spectrally selected by applying a static magnetic fieldB0. (b) Magnetic environment of NV centre electronic spin:13C nuclear spin impurities and N electronic spin impurities. (c) Hahn-echo and multi-pulse (CPMG) spin-control sequences. (d) Negatively charged NV centre electronic energy level structure. Electronic spin polarization and readout is performed by optical excitation at 532 nm and red fluorescence detection. Ground-state spin manipulation is achieved by resonant MW excitation. The ground-state triplet has a zero magnetic field splitting ≈2.87 GHz. Figure 1: NV centre in diamond and applied spin-control pulse sequences. ( a ) Lattice structure of diamond with an NV colour centre. The NV electronic spin axis is defined by nitrogen and vacancy sites, in one of four crystallographic directions in the diamond lattice. NV orientation subsets can be spectrally selected by applying a static magnetic field B 0 . ( b ) Magnetic environment of NV centre electronic spin: 13 C nuclear spin impurities and N electronic spin impurities. ( c ) Hahn-echo and multi-pulse (CPMG) spin-control sequences. ( d ) Negatively charged NV centre electronic energy level structure. Electronic spin polarization and readout is performed by optical excitation at 532 nm and red fluorescence detection. Ground-state spin manipulation is achieved by resonant MW excitation. The ground-state triplet has a zero magnetic field splitting ≈2.87 GHz. Full size image where S ( ω ) is the spectral function describing the coupling of the system to the environment. Equation (1) holds in the approximation of weak coupling of the NV spins to the environment, which is appropriate for systems with (dominantly) electronic spin baths [17] , as is the case with the diamond samples discussed here (see below). S ( ω ) can be determined from straightforward decoherence measurements of the NV spin qubits using a spectral decomposition technique [21] , [22] , [23] . As seen from equation (1), if an appropriate modulation is applied to the NV spins such that , that is, if a Dirac δ -function is localized at a desired frequency ω 0 , then . Therefore, by measuring the time dependence of the qubit coherence C ( t ) when subjected to such a spectral δ -function modulation, we can extract the spin bath's spectral component at frequency ω 0 : This procedure can then be repeated for different values of ω 0 to provide complete spectral decomposition of the spin environment. A close approximation to the ideal spectral filter function F t ( ω ) described above can be provided by a variation on the well-known Carr–Purcell–Meiboom–Gill (CPMG) pulse sequence for dynamical decoupling of a qubit from its environment [27] ( Fig. 1c ). The CPMG pulse sequence is an extension of the Hahn-echo sequence [28] ( Fig. 1c ), with n equally spaced π -pulses applied to the system after initially rotating it into the x axis with a π /2-pulse. We apply a deconvolution procedure to correct for deviations of this filter function from the ideal Dirac δ -function ( Supplementary Fig. S1 and Supplementary Methods ). Spectral function of a spin bath The composite solid-state spin environment in diamond is dominated by a bath of fluctuating N electronic spin ( S =1/2) impurities, which causes decoherence of the probed NV electron-spin qubits through magnetic dipolar interactions. In the regime of low external magnetic fields and room temperature (relevant to the present experiments), the N bath spins are randomly oriented, and their flip-flops (spin-state exchanges) can be considered as random uncorrelated events [17] . Therefore, the resulting spectrum of the N bath's coupling to the NV spins can be assumed to be Lorentzian [25] : This spin-bath spectrum is characterized by two parameters: Δ is the average coupling strength of the N bath to the probed NV spins, and τ c is the correlation time of the N bath spins with each other, which is related to their characteristic flip-flop time. In general, the coupling strength Δ is given by the average dipolar interaction energy between the bath spins and the NV spins, and the correlation time τ c is given by the inverse of the dipolar interaction energy between neighbouring bath-spins. As such spin–spin interactions scale as 1/ r 3 , where r is the distance between spins, it is expected that the coupling strength scales as the N bath spin density n spin (that is, Δ n spin ), and the correlation time scales as the inverse of this density (that is, τ c n spin ). Note also that the multi-pulse CPMG sequence used in the spectral decomposition technique extends the NV spin coherence lifetime by suppressing the time-averaged coupling to the fluctuating spin environment. In general, the coherence lifetime T 2 increases with the number of pulses n used in the CPMG sequence. For a Lorentzian bath, in the limit of very short correlation times ( τ c ≪ T 2 ), the sequence is inefficient and T 2 n 0 (no improvement with number of pulses). In the opposite limit of very long correlation times τ c ≫ T 2 , the scaling is T 2 n 2/3 (refs 29 , 30 , 31 ; see also recent work on quantum dots [32] ). In the following we apply spectral decomposition to study the spin-bath dynamics and resulting scaling of T 2 with n for NV centres in diamond. Experimental application of spectral decomposition The NV centre is composed of a substitutional nitrogen atom and a vacancy on adjacent lattice sites ( Fig. 1a ). The negatively charged state, which is the focus of this work, is believed to gain an electron from nearby nitrogen donor impurities. The energy-level diagram of an NV centre is depicted in Fig. 1d . The NV centre has an electronic spin-triplet ground state with a zero-magnetic-field splitting ≈2.87 GHz between the m s =0 and m s =±1 spin states, quantized along the NV axis. A small external magnetic field applied along this axis lifts the degeneracy of the m s =±1 energy levels with a Zeeman shift ≈2.8 MHz G −1 . Optical transitions between the electronic ground and excited states have a characteristic zero-phonon line at 637 nm, although 532-nm light is typically used to drive excitation to a phonon-sideband, and NV centres fluoresce at room temperature over a broad range of wavelengths that is roughly peaked around 700 nm. Optical cycling transitions between the ground and excited states are primarily spin conserving. However, there exists a decay path that preferentially transfers the m s =±1 excited state population to the m s =0 ground-state through a metastable singlet state, without emitting a photon in the fluorescence band. It is this decay channel that allows the NV centre's spin-state to be determined from the fluorescence signal, and also leads to optical pumping into the m s =0 ground-state. Experimentally, we manipulate the |0 −|1 spin manifold of the NV triplet electronic ground state using a static magnetic field and resonant MW pulses, and use a 532-nm laser to initialize and provide optical readout of the NV spin states ( Fig. 1d ). More specifically, we optically initialize the NV spins to m s =0, apply CPMG pulse sequences ( Fig. 1c ) with varying numbers of π -pulses n and varying free precession times τ , and then measure the NV spin state using optical readout to determine the remaining NV multi-spin coherence (for details see the Methods and refs 13 , 14 , 10 ). The measured coherence is then used to extract the corresponding spin-bath spectral component S n ( ω ) as described above. We applied the spectral decomposition technique to extract the spin-bath parameters Δ and τ c as well as the NV multi-qubit coherence T 2 and FOM for three diamond samples with differing NV densities and concentrations of electronic and nuclear spin impurities ( Table 1 ). The first sample, referred to as the 12 C sample, is an isotopically pure 12 C diamond sample grown by chemical vapour deposition (Element 6), which we studied using an NV wide-field microscope [13] . This sample has a very low concentration of 13 C nuclear spin impurities (0.01%), a moderate concentration of N electronic spin impurities (~1 p.p.m. ), and a moderate NV density (~10 14 (cm −3 )). We then measured the Apollo sample, a chemical vapour deposition diamond sample with a thin N-doped layer with natural 13 C concentration (1.1%), high N concentration (~100 p.p.m. ), and large NV density (~10 16 (cm −3 )), which we also studied using the NV wide-field microscope. The last sample, referred to as the high-pressure high-temperature (HPHT) sample, is a type 1b HPHT diamond sample (Element 6) with natural 13 C concentration, high N concentration (~50 p.p.m.) and low NV density (~10 12 (cm −3 )), which we observed under a confocal microscope able to measure single NV centres. Table 1 Comparison of key characteristics and extracted 'average-fit' Lorentzian spin-bath parameters for the NV-diamond samples studied in this work. Full size table The results for the 12 C sample are summarized in Fig. 2 . In Fig. 2a we plot examples of the measured NV multi-spin coherence decay C n ( t ) as a function of pulse sequence duration t for CPMG pulse sequences with different numbers of π -pulses n . The measured C n ( t ) are well described by a stretched exponential , which is consistent with an electronic spin bath described by a Lorentzian spectrum ( Supplementary Methods ). We analysed such NV decoherence data using the spectral decomposition technique outlined above to extract the best-fit Lorentzian spin-bath spectrum (fit to the average of all data points), yielding a coupling strength of Δ=30±10 kHz and correlation time τ c =10±5 μs, which agrees well with the range of values we find for the Lorentzian spin-bath spectra S n ( ω ) fit to each CPMG pulse sequence individually, Δ 30 to 50 kHz and τ c 5 to 15 μs ( Fig. 2b , see Methods). These values are in reasonable agreement with the expected 'N dominated bath' values for Δ and τ c for this sample's estimated concentrations of 13 C and N spins ( Table 1 ), indicating that N electronic spin impurities are the dominant source of NV decoherence. In Fig. 2c we plot the NV multi-spin coherence lifetime T 2 , determined from the measured coherence decay C n ( t ), as a function of the number n of CPMG π -pulses. 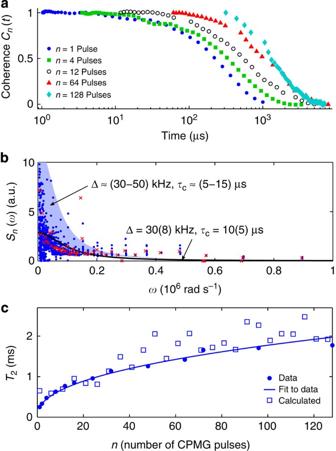Figure 2: Application of the spectral decomposition technique to an isotopically pure12C NV-diamond sample. (a) Examples of measured NV multi-spin coherence as a function of timeCn(t) for CPMG pulse sequences with different numbers of pulsesn. (b) Derived values for the spin-bath spectral functionsSn(ω) for all CPMG pulse sequences (blue dots) and average values at each frequency (red crosses). Each blue dot represents a pulse sequence with a specific durationtand number of pulsesn, such that the probed frequency isω=πn/t. Also shown is the best-fit Lorentzian for the mean spectral functionSn(ω)n(solid black line), and a range of best-fit Lorentzians for the individual spectral functionsSn(ω) for each CPMG pulse sequence (light-blue band); a.u., arbitrary unit. (c) Scaling ofT2with the numbernof CPMG pulses: derived from NV spin coherence decay dataCn(t) (dots); fit of data to a power lawT2=250(40) μs×n0.43(6)(solid line); and synthesized from the average-fit Lorentzian spin-bath spectrum with Δ=30 kHz,τc=10 μs (open squares), which yields a consistent fitT2=270(100) μs×n0.4(1). Figure 2: Application of the spectral decomposition technique to an isotopically pure 12 C NV-diamond sample. ( a ) Examples of measured NV multi-spin coherence as a function of time C n ( t ) for CPMG pulse sequences with different numbers of pulses n . ( b ) Derived values for the spin-bath spectral functions S n ( ω ) for all CPMG pulse sequences (blue dots) and average values at each frequency (red crosses). Each blue dot represents a pulse sequence with a specific duration t and number of pulses n , such that the probed frequency is ω = πn / t . Also shown is the best-fit Lorentzian for the mean spectral function S n ( ω ) n (solid black line), and a range of best-fit Lorentzians for the individual spectral functions S n ( ω ) for each CPMG pulse sequence (light-blue band); a.u., arbitrary unit. ( c ) Scaling of T 2 with the number n of CPMG pulses: derived from NV spin coherence decay data C n ( t ) (dots); fit of data to a power law T 2 =250(40) μs× n 0.43(6) (solid line); and synthesized from the average-fit Lorentzian spin-bath spectrum with Δ=30 kHz, τ c =10 μs (open squares), which yields a consistent fit T 2 =270(100) μs× n 0.4(1) . Full size image We repeated the spectral decomposition analysis for the two other diamond samples, with the results for all three samples summarized in Fig. 3 and Table 1 . We find reasonable agreement between the measured and expected values for the NV/spin-bath coupling strength Δ in all three NV-diamond samples, with Δ scaling approximately linearly with the N concentration. As mentioned before, the measured and expected values for the spin-bath correlation time τ c agree well for the 12 C sample. However, we find a striking discrepancy between the measured and expected values of τ c for the two samples with 1.1% 13 C concentration (Apollo and HPHT): both samples have measured spin-bath correlation times that are more than an order of magnitude longer than that given by the simple electronic spin-bath model, although the relative values of τ c for these two samples scale inversely with N concentration, as expected. 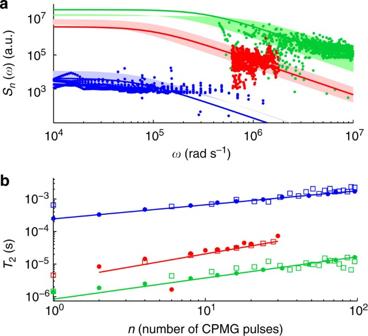Figure 3: Comparative application of the spectral decomposition technique to the12C (blue), Apollo (green) and HPHT (red) NV-diamond samples. (a) Spin-bath spectral functions data for all CPMG pulse sequences (dots), and associated Lorentzian fits using the average-fit method (solid lines) and the individual-fit method (colour bands); a.u., arbitrary unit. (b) Scaling ofT2with the number of CPMG pulsesn: derived from NV spin coherence decay dataCn(t) (dots); fit of dots to a power law (solid lines); and synthesized from the average-fit Lorentzian spin-bath spectrum (open squares). The fitted scalings are:T2n0.43(6)(12C),T2n0.65(5)(Apollo),T2n0.7(1)(HPHT). Figure 3: Comparative application of the spectral decomposition technique to the 12 C (blue), Apollo (green) and HPHT (red) NV-diamond samples. ( a ) Spin-bath spectral functions data for all CPMG pulse sequences (dots), and associated Lorentzian fits using the average-fit method (solid lines) and the individual-fit method (colour bands); a.u., arbitrary unit. ( b ) Scaling of T 2 with the number of CPMG pulses n : derived from NV spin coherence decay data C n ( t ) (dots); fit of dots to a power law (solid lines); and synthesized from the average-fit Lorentzian spin-bath spectrum (open squares). The fitted scalings are: T 2 n 0.43(6) ( 12 C), T 2 n 0.65(5) (Apollo), T 2 n 0.7(1) (HPHT). Full size image We explain this suppression of spin-bath dynamics as a result of random, relative detuning of electronic spin energy levels due to interactions between proximal electronic (N) and nuclear ( 13 C) spin impurities (similar to processes identified by Bloembergen [33] and Portis [34] for other solid-state spin systems). The ensemble average effect of such random electronic-nuclear spin interactions is to induce an inhomogeneous broadening Δ E of the resonant electronic spin transitions in the bath, which reduces the electronic spin flip-flop rate R (~1/ τ c ) given by [35] , [36] where Δ N is the dipolar interaction between N electronic spins. In this physical picture, Δ E is proportional to the concentration of 13 C impurities and to the N- 13 C hyperfine interaction energy, whereas Δ N is proportional to the N concentration. Given the magnetic moments and concentrations of the N and 13 C spin impurities, and the large N– 13 C hyperfine interaction in diamond [37] , [38] , we estimate Δ E ~10 MHz and Δ N ~1 MHz for the Apollo and HPHT samples. These values imply an order of magnitude suppression of R compared with the bare electronic spin flip-flop rate ignoring N– 13 C interactions ( R bare ~Δ N ), which is consistent with our experimental results for τ c ~1/ R ( Table 1 ). The estimate of Δ E is based on a Monte-Carlo simulation of the relative hyperfine interactions of 1,000 N spin pairs with a random distribution of 13 C spin impurities at the natural abundance concentration of 1.1% ( Supplementary Methods ). For the 12 C sample, the low concentration of 13 C spins greatly reduces the magnitude of Δ E , and hence the spin-bath suppression is negligible. Importantly, we found large values for the multi-qubit FOM ~2×10 14 (ms cm −3 ) for both the 12 C and Apollo samples. (The HPHT sample has a relatively low FOM, as expected given its low NV density.) The long coherence time obtained for the Apollo sample, with high NV density, natural 1.1% 13 C abundance and large N concentration, is a result of the combined effect of suppression of electronic spin-bath dynamics and dynamical decoupling: the extended spin-bath correlation time enhances the effectiveness of dynamical decoupling, such that T 2 is increased by a factor of ~10 despite the large concentration of N impurities (which would naively suggest almost no dynamic decoupling improvement of T 2 for this sample [30] ). In summary, we applied the spectral decomposition technique to three NV-diamond samples with different composite-spin environments to characterize the spin-bath dynamics and determine the NV multi-spin-qubit FOM. For samples with a finite concentration of 13 C nuclear spin impurities, this technique revealed an order-of-magnitude suppression of the N electronic spin-bath dynamics, which can be explained by random interactions between proximal electronic and 13 C nuclear spin impurities. This spin-bath suppression enhances the efficacy of dynamical decoupling for samples with high N impurity concentration, enabling increased NV spin coherence times and thus realization of a FOM ~2×10 14 (ms cm −3 ), which is within an order of magnitude of the state-of-the-art spin coherence FOM achieved in atomic systems [15] . Further optimization of the multi-spin-qubit FOM may be possible by engineering this spin-bath suppression, for example, with 13 C concentration higher than the natural value. Such optimization, along with spectral decomposition studies of samples with varying 13 C concentrations, at low temperatures and at high magnetic fields, will be pursued in future work. The present results, together with the possibility of single qubit addressability through AFM [39] , [40] , [41] or super-resolution optical techniques [42] and intrinsic qubit–qubit interactions [1] , pave the way for quantum information, sensing and metrology applications in a robust, multi-qubit solid-state architecture. Finally, the spectral decomposition technique presented here, based on well-known pulse sequences and a simple reconstruction algorithm, can be applied to other composite solid-state spin systems, such as quantum dots and phosphorous donors in silicon. Such measurements could provide a powerful approach for the study of many-body dynamics of complex spin environments, potentially exhibiting non-trivial effects related to the interplay between nuclear and electronic spin baths. Single NV confocal microscope Single NV measurements (HPHT sample) were performed using a custom-built confocal microscope. Optical excitation was provided by a 300 mW 532 nm diode pumped solid-state laser (Changchun New Industries Optoelectronics Tech, MLLIII532-300-1), focused onto the sample using a ×100, NA=1.3 oil-immersion objective (Nikon CFI Plan Fluor ×100 oil). NV fluorescence was collected through the same optics, and separated from the excitation beam using a dichroic filter (Semrock LM01-552-25). The light was additionally filtered (Semrock LP02-633RS-25) and focused onto a single-photon counting module (Perkin-Elmer, SPCM-ARQH-12). The excitation laser was pulsed by focusing it through an acousto-optic modulator (Isomet 1205C-2). Microwaves were delivered to the sample through a 20-μm thick wire soldered across it. The wire was driven by an amplified (Mini-circuits ZHL-16W-43-S+) MW synthesizer (Agilent E4428C). Phase modulation of the MW pulses was achieved using an in-phase/quadrature (IQ) mixer (Marki IQ-1545). MW and optical pulses were controlled using a computer-based digital delay generator (SpinCore PulseBlaster ESR400). A static magnetic field of ≈50 G was applied to the sample to lift the degeneracy of the m s =±1 levels. NV wide-field fluorescence microscope NV multi-spin measurements (for samples 12 C and Apollo) were performed using a custom-built wide-field fluorescence microscope ( Fig. 4a ), which has previously been used for two-dimensional magnetic field imaging with thin-layer NV-diamond samples [13] . Optical excitation was provided by a 3-W 532-nm laser (Laser Quantum Opus), which illuminated a large region of interest on the diamond surface through a ×20 NA=0.75 objective (Nikon). An acousto-optic modulator (Isomet M1133-aQ80 L-H) acted as an optical switch, to pulse the laser with precise timing in order to prepare and detect the NV spin states. A loop antenna was positioned near the diamond surface and connected to the amplified (Mini-circuits ZHL-16W-43-S+) output of a microwave signal generator (Agilent E8257D) to generate a homogeneous B 1 field over the region of interest. Fast-switching of the MW field (ZASWA-2-50DR) enabled coherent manipulation of the NV spin states necessary for coherence decay measurements using CPMG pulse sequences, in order to perform the spectral decomposition technique. Optical and MW pulse timings were controlled through a computer-based digital delay generator (SpinCore PulseBlaster PRO ESR500). 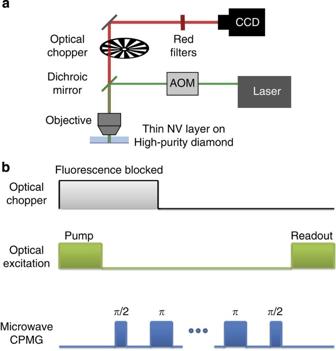Figure 4: Details of ensemble measurement setup and pulse sequences. (a) Diagram of the NV wide-field fluorescence microscope. The laser produces 532-nm light, which is switched by the acousto-optic modulator (AOM) and directed through a dichroic mirror and an objective onto the diamond sample. The fluorescence from the sample passes through the dichroic and, following an optical chopper and appropriate filters, is collected by a charge-coupled device (CCD). (b) Pulse sequence used to perform spectral decomposition measurements with the NV wide-field microscope. Optical pulses are used to first initialize the NV and then to readout its spin state. The optical chopper is synced such that the initialization pulse is blocked from the CCD, while the readout pulse is recorded. The microwave pulses are applied between the initialization and readout optical pulses. Figure 4: Details of ensemble measurement setup and pulse sequences. ( a ) Diagram of the NV wide-field fluorescence microscope. The laser produces 532-nm light, which is switched by the acousto-optic modulator (AOM) and directed through a dichroic mirror and an objective onto the diamond sample. The fluorescence from the sample passes through the dichroic and, following an optical chopper and appropriate filters, is collected by a charge-coupled device (CCD). ( b ) Pulse sequence used to perform spectral decomposition measurements with the NV wide-field microscope. Optical pulses are used to first initialize the NV and then to readout its spin state. The optical chopper is synced such that the initialization pulse is blocked from the CCD, while the readout pulse is recorded. The microwave pulses are applied between the initialization and readout optical pulses. Full size image NV fluorescence was collected by the objective, filtered, and imaged onto a cooled charge-coupled device camera (Starlight Xpress SXV-H9). As the duration of a single measurement is shorter than the minimum exposure time of the camera, the measurement was repeated for several thousand averages within a single exposure and synchronized to an optical chopper placed before the camera in order to block fluorescence from the optical preparation pulse ( Fig. 4b ). Repeating the measurement without the MW control pulses provided a reference for long-term drifts in the fluorescence intensity. In the measurements described here, the loop of wire delivered 3.07 GHz MW pulses to the sample, resonant with the NV |0 −|1 spin transition for the applied static magnetic field ≈70 G, to manipulate the NV spin coherence and implement CPMG spin-control pulse sequences. Spectral decomposition deconvolution procedure The coherence of a two-level quantum system can be related to the magnitude of the off-diagonal elements of the system's density matrix. Specifically, we deal here with NV electronic spin qubits in a finite external magnetic field, which can be treated as effective two-level spin systems with quantization ( z ) axis aligned with the NV axis. When the NV spins are placed into a coherent superposition of spin eigenstates, for example, aligned with the x axis of the Bloch sphere, the measurable spin coherence is given by . The filter function for the n -pulse CPMG control sequence F CPMG ( ω ) covers a narrow frequency region (given by π / t , where t is total length of the sequence), which is centred at ω 0 = πn/t , and is given by [43] : We note that the narrow-band feature of the CPMG filter essentially defines the effectiveness of this sequence for dynamical decoupling. The filter function associated with the CPMG pulse sequence deviates from a δ -function by the finite width of the main spectral peak and by the presence of higher harmonics ( Supplementary Fig. 1 ). In addition, the central frequency of the filter function changes with the duration of the experiment and with the number of pulses. Therefore, reconstructing the spin-bath spectral function S ( ω ) from the decoherence data requires a solution of the Fredholm type equation to extract S ( ω ) equation (1): This extraction is accomplished by assuming that the spectral function decays to zero at high frequency and by noting that the filter function includes high harmonics but negligible low frequency artefacts. Thus, the procedure starts at the high frequency values of C ( ω ), and works back to lower frequencies by subtracting the effect of higher harmonics using the reconstructed high frequency values of S ( ω ) and the analytical form of the filter function. Owing to the high frequency components of the filter function and the monotonically decreasing nature of the spectral function, a naive reconstruction of the spectral function assuming a δ -function form of the filter function produces results that are biased to lower values by ~15%. This bias is removed using the reconstruction algorithm presented above. How to cite this article: Bar-Gill, N. et al . Suppression of spin-bath dynamics for improved coherence of multi-spin-qubit systems. Nat. Commun. 3:858 doi: 10.1038/ncomms1856 (2012).